Virtual hyperbolic metamaterials for manipulating radar signals in air Microwave beam transmission and manipulation in the atmosphere is an important but difficult task. One of the major challenges in transmitting and routing microwaves in air is unavoidable divergence because of diffraction. Here we introduce and design virtual hyperbolic metamaterials (VHMMs) formed by an array of plasma channels in air as a result of self-focusing of an intense laser pulse, and show that such structure can be used to manipulate microwave beams in air. Hyperbolic, or indefinite, metamaterials are photonic structures that possess permittivity and/or permeability tensor elements of opposite sign with respect to one another along principal axes, resulting in a strong anisotropy. Our proof-of-concept results confirm that the proposed virtual hyperbolic metamaterial structure can be used for efficient beam collimation and for guiding radar signals around obstacles, opening a new paradigm for electromagnetic wave manipulation in air. When microwaves or terahertz beams propagate in air, they diffract, as does any electromagnetic beam. Therefore, to be able to receive a signal of appreciable intensity at a distance, one has to either increase the intensity of the incident beam or counteract this beam-broadening diffraction effect. Moreover, detection of radar signals in a realistic environment may be negatively affected by the divergence of the beam resulting from distortions by natural obstacles, for example, by non-planar landscapes. To overcome the distortion of beams propagating in such environments, some method of guiding the beam around obstacles (or ‘cloaking’ the obstacles) is desirable. The development of ordered structures of laser-induced plasma filaments opens the possibility of creating conductive filamentary structures capable of guiding microwaves or terahertz frequency radiation. In the last few years, various types of filament-based waveguides (conducting or dielectric like) have been proposed for channelling microwaves [1] , [2] , [3] , [4] , [5] . Guiding of 10 GHz radiation with filaments was experimentally demonstrated by Chateauneuf et al . [3] using a 100 TW laser system to produce a cylindrical array 45 mm in diameter composed of ~1,000 filaments. A 10-GHz signal was coupled into the induced plasma waveguide and guided over a distance of 16 cm. The intensity of the guided signal detected at the exit of the cylindrical array was increased by a factor greater than six compared with the free propagation of the microwave radiation. Although this approach offers a way to counteract the diffraction of a radar signal over some distance, the issues of beam steering and coupling microwave signals into such waveguides are likely to be challenging. Finally, very recently, Marian et al . [6] reported parametric studies of interactions of microwaves with subwavelength arrays of parallel plasma filaments. Although these studies elucidated reflection and transmission properties of various periodically and randomly arranged filament arrays, no specific physical mechanism enabling guiding, focusing or steering of the microwave beam was discussed. In this Article, we propose a fundamentally new approach based on unique physical properties of virtual hyperbolic metamaterials (VHMMs) formed of plasma filaments in air. We show that VHMMs can be used for focusing, guiding and steering radar signals to facilitate new degrees of freedom in the detection of such signals in realistic environments. Further, we show that by variation of realistically available parameters of VHMM, such as fill-fraction of plasma filaments and recombination rate of free electrons with positive ions inside the filament channels (that can be controlled by heat), it is possible to control the performance of the VHMM structure. Mathematical model of VHMMs Consider a microwave beam incident on a two-dimensional rectangular array of filaments or microscopic wires of conductivity, as shown in Fig. 1a . 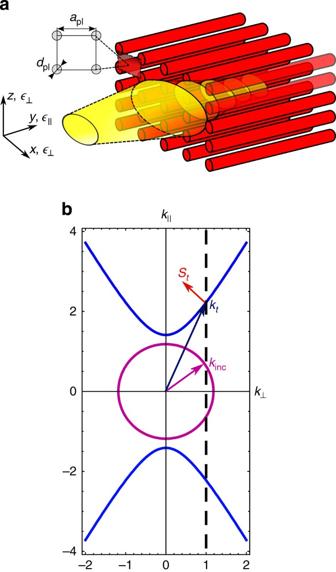Figure 1: Concept of the VHMM. (a) Schematic illustration of the filament-based VHMM formed of laser-induced plasma filaments (red wires) in air for microwave signal guiding (schematically shown as yellow trace of the beam). The lower inset shows the orientation of the coordinate system and corresponding component of the permittivity tensorε||andε⊥. The upper inset outlines two characteristic geometrical parameters of VHMM diameter of plasma channel (dpl) and distance between filaments (apl); (b) Isofrequency contour for free space (circular) and VHMM (hyperbolic). Figure 1b shows isofrequency curves and relative directions of the Poynting vector S and wave vector k . In the isotropic case, the isofrequency surfaces are circles and, therefore, S ∇ k ω ( k ) k (that is, vectors S and k are collinear), whereas in anisotropic materials the wave vector surfaces become either ellipsoidal or hyperbolic, depending on the signs of ε ⊥ and ε || . Taking y as the direction of the optical axis, we can characterize the extraordinary wave in a uniaxial anisotropic structure by the dispersion relation Figure 1: Concept of the VHMM. ( a ) Schematic illustration of the filament-based VHMM formed of laser-induced plasma filaments (red wires) in air for microwave signal guiding (schematically shown as yellow trace of the beam). The lower inset shows the orientation of the coordinate system and corresponding component of the permittivity tensor ε || and ε ⊥ . The upper inset outlines two characteristic geometrical parameters of VHMM diameter of plasma channel ( d pl ) and distance between filaments ( a pl ); ( b ) Isofrequency contour for free space (circular) and VHMM (hyperbolic). Full size image where ε || and ε ⊥ are the components of the dielectric permittivity tensor parallel to the wires and perpendicular to the wires, respectively, k || and k ⊥ are corresponding components of the wave vector, ω is the angular frequency and c is the speed of light. In the case of hyperbolic metamaterials, the components of dielectric permittivity satisfy the following condition: ε ⊥ >0, ε || <0 and the signs of the projections of S t and k t on to the x axis are opposite. As a result, such structures support negative refraction and can be used for focusing and steering electromagnetic radiation [7] , [8] , [9] , [10] , [11] , [12] , [13] , [14] , [15] . Conventionally, hyperbolic metamaterials are realized using either metal/dielectric multilayers or an array of metal wires in a dielectric matrix [10] , [11] , [12] , [13] , [14] , [15] . Here we show that an array of plasma filaments formed by the propagation of intense short pulses in air is able to form a VHMM structure. Indeed, plasma filaments have the role of metal wires and the air has the role of a dielectric host. We propose to use hyperbolic metamaterial-like structures formed from filaments in air, with approximate diameters d pl ≈50~120 μm (ref. 1 ) and average distance between filaments a pl ≈450~650 μm for microwave and terahertz guiding ( Fig. 1a ). If the wavelength of the incident electromagnetic (EM) field λ inc is much larger than the diameter d pl , the EM wave cannot resolve individual filaments, and the composite medium can be considered as an effective medium. The two components of the permittivity tensor, perpendicular to direction of propagation ( ε ⊥ ) and parallel to the direction of propagation ( ε || ), can be calculated using the mixing rule as [12] where f is the fill-fraction of filaments ( f = d pl / a pl in the two-dimensional case and in the three-dimensional case); ε air and ε fil ( ω ) are the permittivities of the air and filament channel, respectively. The permittivity of the filament channel can be described by the Drude model as where is the plasma frequency, e and m e are the electron charge and mass, respectively, ε 0 is the permittivity of free space, N e is the electron density and ν is the collision frequency. The concentration of the electrons inside the laser-induced filament channel in air varies between 10 15 and 10 17 cm −3 (refs 1 , 5 ) and the corresponding plasma frequency range is 300–3,000 GHz (ref. 5 ). Generally, for plasma filaments in the air, where the gas is not fully ionized, the collision frequency is given by where is an electron-ion collision frequency, T e is the electron temperature, (ln Λ) is Coulomb logarithm, is an electron-neutral collision frequency and N a is the density of the atoms. In the case of weakly ionized gas at a pressure of 1 atm, N e =10 17 cm −3 , T e =1 eV, N a =2.7 × 10 19 cm −3 , the collision frequency [4] is ν ei ≈7.61 × 10 10 s −1 and ν en ≈1.05 × 10 12 s −1 . The dynamics of the electron density ( N e ), the density of positive ( N + ) and negative ions ( N − ) inside each filament can be calculated using rate equations [16] , [17] where α is the collisional ionization rate, η is the attachment rate, β e+ is the electron-positive ion recombination rate coefficient and β −+ is the recombination rate coefficient between negative ions and positive ions. In the case of atmospheric pressure and in the absence of any external fields, the collisional ionization rate ( α ) is much smaller than the attachment rate coefficient ( η ), and thus can be neglected ( α ≈0). At the same time, electrons participate in three-body reaction with rate η 3 and two-body reaction with rate η 2 , which leads to the creation of negative molecular ions ( ) and negative ions (O − ), respectively. Therefore, the total attachment rate coefficient [18] , [19] is η = η 2 + η 3 ≈2.5 × 10 7 s −1 . Another important phenomenon, which takes place inside the filament channel, is the recombination between electrons and positive ions, and similarly between negative ions with positive ions, with corresponding rate coefficients β e+ and β −+ . Recombination rate coefficients are defined as and β −+ ≈2.2 × 10 −13 m 3 s −1 (ref. 19 ). The system of rate equation (5) is solved numerically with the assumptions that initial N e = N + ≈2 × 10 17 cm −3 , N − ≈0. 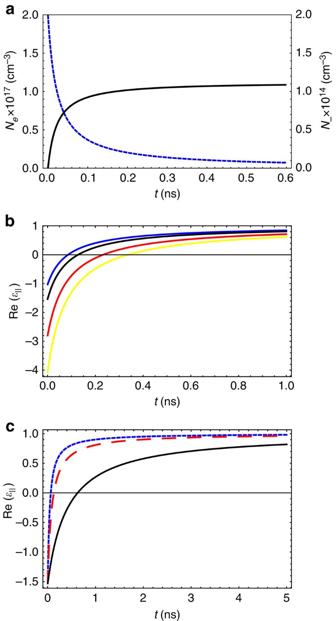Figure 2: Density and permittivity of the VHMM. (a) Evolution of electron (dashed blue curve) and negative ion (solid black curve) densities inside filament channels; (b) Real part ofε||as a function of time for different fill-fraction of filamentsf=0.08 (blue curve),f=0.1 (black curve),f=0.15 (red curve) andf=0.2 (yellow curve), and fixed recombination rate coefficientβe+=1.2 × 10−13m3s−1; (c) Real part ofε||as a function of time for different recombination rate coefficientsβe+=1.2 × 10−13m3s−1(dotted blue curve),βe+=0.6 × 10−13m3s−1(dashed red curve) andβe+=0.12 × 10−13m3s−1(solid black curve), and fixed fill-fractionf=0.1. Figure 2a shows the evolution of electron, positive and negative ions densities inside filament channels with time. Reduction of the electron density of filaments with time results in the VHMM medium having time-dependent effective permittivity. Figure 2b shows the real part of ε || as a function of time for the fill-fraction of filaments, which varies from 0.08 to 0.2. It is noteworthy that the real part of ε || changes sign when a particular moment in time is reached, whereas the real part of ε ⊥ remains positive and, for example, for f =0.1 equals Re( ε ⊥ )=1.2. As a result, the dispersion relation of the VHMM changes from hyperbolic to elliptical when ε || becomes positive. As long as the dispersion relation remains hyperbolic, the diverging Gaussian beam entering from air to VHMM is negatively refracted and converging/collimated inside the effective medium, assuming it did not reach its focus point. Figure 2b indicates that the higher the fill-fraction, the longer ε || stays negative, that is, the dispersion relation remains hyperbolic. Figure 2: Density and permittivity of the VHMM. ( a ) Evolution of electron (dashed blue curve) and negative ion (solid black curve) densities inside filament channels; ( b ) Real part of ε || as a function of time for different fill-fraction of filaments f =0.08 (blue curve), f =0.1 (black curve), f =0.15 (red curve) and f =0.2 (yellow curve), and fixed recombination rate coefficient β e+ =1.2 × 10 −13 m 3 s −1 ; ( c ) Real part of ε || as a function of time for different recombination rate coefficients β e+ =1.2 × 10 −13 m 3 s −1 (dotted blue curve), β e+ =0.6 × 10 −13 m 3 s −1 (dashed red curve) and β e+ =0.12 × 10 −13 m 3 s −1 (solid black curve), and fixed fill-fraction f =0.1. Full size image Microwave signal guiding and steering using VHMM Once the effective permittivity tensor is determined using equations (2)–(5), we investigate the propagation of the microwave beam inside the VHMM medium using Maxwell’s equations The relative permeability of the medium μ is assumed to be equal to one. Noting that the incident field is assumed to be a transverse-magnetic (TM) polarized continuous wave Gaussian beam with a wavelength λ inc =5 cm, the components of the incident EM wave are chosen as H ={0,0, H z } and E ={ E x , E y ,0}. Here we summarize several assumptions that have been made. As we consider the VHMM structure made of plasma filaments with initial free electron density 2 × 10 17 cm −3 and fill-fraction f =0.1, in reality it is difficult to achieve this configuration without any background plasma between the filaments. We neglect the background plasma in the simulations, and assume that VHMM consists of plasma filaments and air (see equation (2)). Besides, it is a well-known fact that it is difficult to achieve plasma filaments with such configuration (electron density and fill-fraction) longer than few centimetres in air. Within this work, we make an assumption that VHMM structure can be of arbitrary length and the guiding of the signal wave is limited only by the lifetime of the plasma filaments inside VHMM medium. On the basis of developed finite-difference time domain (FDTD) code [20] , we have considered the case when microwave signal propagates in the free space (negative values of y axis) and launches to VHMM medium (positive values of y axis), while the air-VHMM boundary is set to be at the point y =0 (see Fig. 3 ). Besides this, we need to mention that at the initial moment of time (first 0.3 ns) while the microwave signal propagates inside the free space, the components of the dielectric permittivity tensor( ε ⊥ and ε || ) are assumed to be constant and determined by initial concentration of free electrons inside plasma filaments N e (0). The components of the dielectric permittivity tensor ( ε ⊥ and ε || ) are considered to be time dependent once the microwave beam reaches the air-VHMM boundary. This assumption implies negligibly small time delay between high-power excitation laser, which forms VHMM structure, and microwave signal. 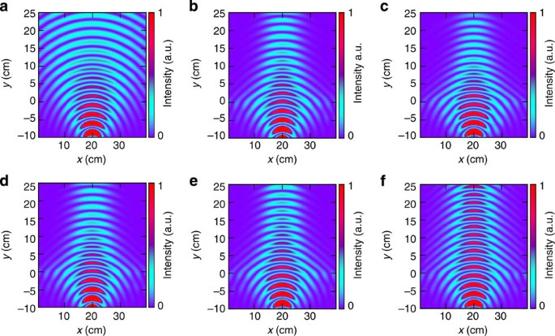Figure 3: Intensity distributions forλ=5 cm. The field intensity distribution for TM-polarized continuous wave Gaussian beam at wavelengthλ=5 cm propagating in (a) air, (b) in a VHMM with fill-fractionf=0.1 and (c) in a VHMM withf=0.2, and for fixed fill-fractionf=0.1 but different recombination rate coefficients (d)βe+=1.2 × 10−13m3s−1, (e)βe+=0.6 × 10−13m3s−1and (f)βe+=0.12 × 10−13m3s−1. Figure 3: Intensity distributions for λ =5 cm. The field intensity distribution for TM-polarized continuous wave Gaussian beam at wavelength λ =5 cm propagating in ( a ) air, ( b ) in a VHMM with fill-fraction f =0.1 and ( c ) in a VHMM with f =0.2, and for fixed fill-fraction f =0.1 but different recombination rate coefficients ( d ) β e+ =1.2 × 10 −13 m 3 s −1 , ( e ) β e+ =0.6 × 10 −13 m 3 s −1 and ( f ) β e+ =0.12 × 10 −13 m 3 s −1 . Full size image Figure 3 shows the intensity distribution for three cases: air ( Fig. 3a ), VHMM with fill-fraction f =0.1 ( Fig. 3b ) and VHMM with fill-fraction f =0.2 ( Fig. 3c ) at t =1.2 ns moment of time. Figures 3b,c confirm the prediction that the VHMM structure can be used to compensate for strong diffraction broadening of a microwave beam propagating in a free space. It clearly shows that a larger fill-fraction of filaments leads to a stronger focusing effect in the beam. At the same time, it should be noted that a microwave beam propagating in a VHMM experiences losses associated with the metallic nature of plasma filaments, and as a result, the beam intensity decays with propagation distance. It should also be noted that the decay of plasmas in the wake of the laser pulse limits the lifetime of plasma-induced filament-array waveguides. Fortunately, it was proposed and demonstrated that the lifetime of the filaments can be increased by heating plasma filaments with a second, delayed nanosecond pulse [21] , [22] or by employing a system composed of a dual femtosecond/nanosecond laser pulse [23] , [24] . Such additional delayed laser pulses efficiently increase electron temperature, and as a result, suppress dissociative recombination. Therefore, we performed a study of microwave propagation in a VHMM for different recombination rate coefficient β e+ , as shown in Fig. 3d–f . Figure 3d shows microwave beam propagation corresponding to the no-heating case with β e+ =1.2 × 10 −13 m 3 s −1 and f =0.1. Figure 3e,f shows the cases corresponding to β e+ =0.6 × 10 −13 m 3 s −1 and β e+ =0.12 × 10 −13 m 3 s −1 , respectively, for the same fill-fraction f =0.1. These results clearly indicate that decreasing the recombination rate would significantly increase the distance of microwave beam guiding by VHMM. To quantify the improvement in microwave guidance enabled by VHMM, we calculate transmission enhancement factor ζ = I VHMM / I air as a ratio of on-axis peak time average intensities of the signal transmitted through focusing VHMM medium ( I VHMM ) and of the signal propagating in a free space ( I air ). Transmission enhancement factor is calculated and studied only for positive values of y . 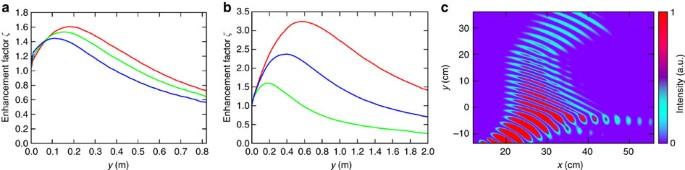Figure 4: Enhancement factors. Transmission enhancement factorζ=IVHMM/Iairas a function of propagation distance for different fill-fractions:f=0.1 (red curve),f=0.15 (green curve) andf=0.2 (blue curve;a). Transmission enhancement factorζ=IVHMM/Iairas a function of propagation distance for different recombination rates:βe+=1.2 × 10−13m3s−1(green curve),βe+=0.6 × 10−13m3s−1(blue curve) andβe+=0.12 × 10−13m3s−1(red curve;b). (c) Beam steering using VHMMs (f=0.1 andβe+=0.12 × 10−13m3s−1). Figure 4a shows the transmission enhancement factor ζ as a function of propagation distance for different fill-fractions of filaments. As discussed above, inside the VHMM, an initially diverging microwave beam experiences a focusing effect, whereas the same beam propagating in a free space diverges because of diffraction. Accordingly, the enhancement factor ζ increases. However, it can be seen in Fig. 4a that after a certain propagation distance, losses inside the VHMM become significant, leading to reduction of the transmission enhancement factor. This suggests that the design of the VHMM can be optimized for the desired propagation distance and enhancement factor. For example, propagation distance corresponding to ζ =1 and to I VHMM = I air ranges from 0.3 to 0.5 m for different fill-fraction parameters. Figure 4b shows the transmission enhancement factor ζ as a function of propagation distance for different recombination rates, demonstrating that both the enhancement factor and the distance corresponding to the maximum enhancement increase as recombination rate coefficient decreases. These results are in agreement with the prediction of Fig. 3d,f . Figure 4: Enhancement factors. Transmission enhancement factor ζ = I VHMM / I air as a function of propagation distance for different fill-fractions: f =0.1 (red curve), f =0.15 (green curve) and f =0.2 (blue curve; a ). Transmission enhancement factor ζ = I VHMM / I air as a function of propagation distance for different recombination rates: β e+ =1.2 × 10 −13 m 3 s −1 (green curve), β e + =0.6 × 10 −13 m 3 s −1 (blue curve) and β e+ =0.12 × 10 −13 m 3 s −1 (red curve; b ). ( c ) Beam steering using VHMMs ( f =0.1 and β e+ =0.12 × 10 −13 m 3 s −1 ). Full size image Finally, Fig. 4c demonstrates another potentially useful functionality—microwave beam steering enabled by filament-based VHMM in air. In this case, the VHMM structure is formed such that the microwave beam enters the VHMM at an angle. The angle of refraction can be controlled by changing the fill-fraction of the filaments. It is noteworthy that the microwave beam refracts negatively with respect to the normal to the air-VHMM interface. Such negative refraction is again due to hyperbolic dispersion relations. Indeed, it can be seen in Fig. 1b that the projections of the Poynting vector S and wave vector k on the horizontal axis ( k ⊥ ) are antiparallel, resulting in such negative refraction, as shown in Fig. 4c . We envision that such reconfigurable engineered VHMM-based beam steering ‘devices’ will be useful in natural environments where the detection of radar signals may be complicated by divergence of the beam during its free space propagation or because of distortions by various obstacles. It is noteworthy that the proposed approach of guiding microwave beams using the VHMMs is robust with respect to changes in the filaments parameters, and the wavelength of the microwave radiation and in general does not require rather high free electron densities and it can realized at lower free electron densities than those considered above. Here we show that similar performance can be achieved at lower free electron densities, for example, n e =5 × 10 16 cm −3 , and at a different microwave wavelength λ =7.5 cm. 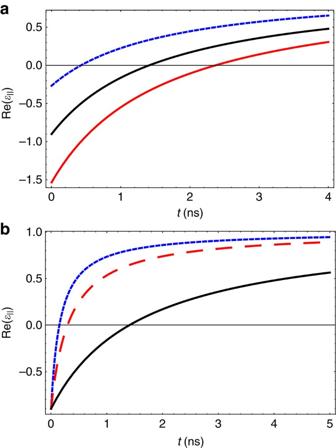Figure 5: Permittivity behaviour. (a) Real part ofε||as a function of time for different fill-fraction of filamentsf=0.2 (dotted blue curve),f=0.3 (solid black curve) andf=0.4 (solid red curve), and fixed recombination rate coefficientβe+=1.2 × 10−13m3s−1. (b) Real part ofε||as a function of time for different recombination rate coefficientsβe+=1.2 × 10−13m3s−1(dotted blue curve),βe+=0.6 × 10−13m3s−1(dashed red curve) andβe+=0.12 × 10−13m3s−1(solid black curve) and fixed fill-fractionf=0.3. Figure 5a shows real part of ε || as a function of time for different fill-fraction of filaments at a fixed recombination rate coefficient. Figure 5b shows real part of ε || as a function of time for different recombination rate coefficients at a fixed fill-fraction f =0.3. Finally, Fig. 6 shows field intensity distributions for a TM-polarized continuous wave Gaussian beam at wavelength λ =7.5 cm in VHMMs with different fill-fraction for given recombination rate coefficient β e+ =0.12 × 10 −13 m 3 s −1 . Figure 5: Permittivity behaviour. ( a ) Real part of ε || as a function of time for different fill-fraction of filaments f =0.2 (dotted blue curve), f =0.3 (solid black curve) and f =0.4 (solid red curve), and fixed recombination rate coefficient β e+ =1.2 × 10 −13 m 3 s −1 . ( b ) Real part of ε || as a function of time for different recombination rate coefficients β e+ =1.2 × 10 −13 m 3 s −1 (dotted blue curve), β e+ =0.6 × 10 −13 m 3 s −1 (dashed red curve) and β e+ =0.12 × 10 −13 m 3 s −1 (solid black curve) and fixed fill-fraction f =0.3. 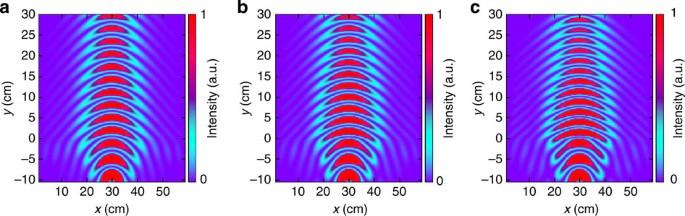Figure 6: Intensity distributions forλ=7.5 cm. Field intensity distributions for a TM-polarized continuous wave Gaussian beam at wavelengthλ=7.5 cm in (a) vHMM with fill-fractionf=0.2; (b) VHMM with fill-fractionf=0.3; and (c) vHMM with fill-fractionf=0.4 for given recombination rate coefficientβe+=0.12 × 10−13m3s−1. Full size image Figure 6: Intensity distributions for λ =7.5 cm. Field intensity distributions for a TM-polarized continuous wave Gaussian beam at wavelength λ =7.5 cm in ( a ) vHMM with fill-fraction f =0.2; ( b ) VHMM with fill-fraction f =0.3; and ( c ) vHMM with fill-fraction f =0.4 for given recombination rate coefficient β e+ =0.12 × 10 −13 m 3 s −1 . Full size image In summary, in this paper we proposed to use VHMMs formed by an array of plasma channels in air to manipulate microwave radar signals. We performed a comprehensive study of the performance of such VHMMs and demonstrated that using various realistically available degrees of freedom such as fill-fraction of plasma filaments and recombination rate (that can be controlled by heat), one can remotely focus, guide and steer radar signals to facilitate new degrees of freedom in the detection of such signals in realistic environments. Solution of the Maxwell equation for VHMM structure The system of Maxwell’s equations: is solved numerically using the FDTD method within the auxiliary differential equation (ADE) technique. By taking into account equation(2), the material equation for electric displacement field D for different component of the field can be rewritten in the following way: where permittivity of the filaments is determined by the Drude model. By implementing inverse Fourier transform of equation (8), the ADEs, which determine relation between components of electric field E and corresponding components of electric displacement field D in time domain, can be derived. The ADE in the case under consideration takes the following form: here g 1 =(1– f )+(1+ f ) ε air , g 2 =1+ f +(1– f ) ε air . To determine spatial distribution of the E and H field at the given moment of time, the system of curl equations from equation (7) and one of the ADE (equation (9)) for corresponding field component should be solved simultaneously. For the case of TM incident wave for each time step, the following equations should be solved: To determine E x : To determine E y : For determine H z : It is noteworthy that plasma frequency ω p in equation (9) in the case under consideration is a time-dependent parameter because of evolution of the free electron concentration inside the filaments and need to be updated at every time step. The system equations(10)–(12), is solved with help of leapfrog scheme within FDTD technique. [20] , [25] How to cite this article: Kudyshev, Z. A. et al . Virtual hyperbolic metamaterials for manipulating radar signals in air. Nat. Commun. 4:2557 doi: 10.1038/ncomms3557 (2013).